A fast and unbiased procedure to randomize ecological binary matrices with fixed row and column totals A well-known problem in numerical ecology is how to recombine presence-absence matrices without altering row and column totals. A few solutions have been proposed, but all of them present some issues in terms of statistical robustness (that is, their capability to generate different matrix configurations with the same probability) and their performance (that is, the computational effort that they require to generate a null matrix). Here we introduce the ‘Curveball algorithm’, a new procedure that differs from existing methods in that it focuses rather on matrix information content than on matrix structure. We demonstrate that the algorithm can sample uniformly the set of all possible matrix configurations requiring a computational effort orders of magnitude lower than that required by available methods, making it possible to easily randomize matrices larger than 10 8 cells. Many ecological patterns are investigated by analysing presence-absence (1-0) matrices [1] . This holds both for matrices describing distribution of taxonomic units (that is, species per site matrices) and for matrices describing species interactions (that is, ecological network matrices) [2] . Species co-occurrence, nestedness and modularity (that is, the non-random occurrence of densely connected, non-overlapping species subsets) are typical examples of matrix analyses used in community ecology, biogeography, conservation, and host-parasite interaction studies [3] . Although several metrics have been proposed to quantify peculiar matrix aspects, none of them has associated probability levels. Thus, comparing the patterns found in a given matrix with those emerging from randomly generated matrices (null models) is a common procedure to assess the probability that the observed pattern can be explained by chance alone [4] . For this, the matrix under study is randomized several times, and the pattern observed in the original matrix is compared with the patterns observed in the random matrices. In doing this, however, the choice of the ‘rules’ controlling the randomization process may lead to very different outcomes, thus making the interpretation of results difficult [5] . This happens because null models may vary a lot in their restrictiveness; that is, in how much a null matrix preserves features of the original matrix [6] . Some basic matrix properties, such as size (that is, number of matrix cells) and fill (that is, the ratio between number of occurrences and matrix size) are commonly retained in the generation of null matrices even by the least restrictive null models [5] and several studies highlight the importance of generating null matrices with the same row and column totals as those of the matrix under study to minimize the risk of type II errors [5] , [7] . Moreover, preserving row and column totals has deep ecological implications [2] . For example, in a species per site matrix, a row with several presences may suggest that the corresponding species, which occurs in several localities, is an ecological generalist. On the other hand, a column with many presences may indicate that the considered locality, which is inhabited by several different species, has a high resource availability. Thus, preserving row and column totals should be preferable in most situations [2] , [8] , [9] , and especially in the analysis of species co-occurrence [4] . However, generating random matrices that preserve row and column totals is far from trivial. Several statistical approaches have been proposed to this purpose [10] , [11] , [12] , [13] , [14] . Most of them use algorithms based on swaps of ‘checkerboard units’ [13] , where a checkerboard unit [15] is a 2 × 2 submatrix in one of the two alternative configurations: Swap methods, at each cycle, extract at random two rows and two columns from the matrix. If the 2 × 2 submatrix including the cells at the intersection of these rows and columns is a checkerboard unit, it is swapped, that is, the values of one of its diagonal are replaced with the values of the other one (thus passing from one checkerboard configuration to another one). The most commonly used swap algorithm is the ‘sequential swap’, which generates a first null matrix by performing 30,000 swaps, and then creates each subsequent null matrix by performing a single swap on the last generated matrix [13] . As a consequence, independent of the number of swaps performed, each matrix in the resulting set differs from the previous one by only four matrix elements. Thus, to create a set of matrices truly representative of the whole set of possible configurations, a very large number of null matrices must be generated [16] , [17] . Alternatively, one may use the independent swap algorithm, which creates each null matrix by performing a certain number of swaps (ideally more than 30,000) on the original matrix [13] , [18] . However, swap methods tend to be biased towards the construction of segregated matrices, that is, matrices with more checkerboard units than expected by chance [14] . Thus none of these approaches (that is, generating a large number of null matrices, or using the independent swap algorithm) guarantees that the set of null matrices generated constitutes a truly random sample of the universe of possible matrix configurations [13] . A different method, based on random walks on graphs, has been demonstrated to be unbiased [19] . However, this approach, which was primarily conceived as an aid for testing biogeographical hypotheses, has rarely been applied to practical ecological studies, perhaps as a consequence of its complexity. A simpler algorithm is the ‘trial-swap’ [14] , which consists a subtle modification of the traditional swap algorithms, based on the principle of setting a priori the number of total swaps to be attempted on a matrix. The trial-swap algorithm samples different null matrices with the same probability. Yet, since the convergence to the uniform distribution of null matrices may be slow (that is, it may require many swaps) for large data sets, this algorithm should be combined with two much faster algorithms that, however, have not been proven to lead to the uniform distribution. Thus, faster algorithms are used to create a first null matrix and the trial-swap algorithm is used in subsequent perturbations to generate the uniform distribution of results [14] , [20] . Other authors suggested using the sequential swap and correcting it for unequal frequencies [16] , [19] . More recently, an efficient algorithm for sampling exactly from the uniform distribution over binary or non-negative integer matrices with fixed row and column sums was developed [21] . However, this method can be applied only to small matrices (with a total number of rows and columns less than 100) or larger matrices with low fill [21] . Thus, despite the higher statistical robustness of some of the above-mentioned procedures, the sequential swap still remains the most commonly used algorithm to generate null matrices with fixed row and column totals [17] . Here we show how a childhood pastime such as trading baseball cards may suggest an alternative and effective solution to the problem of presence-absence matrix permutations, by introducing a new algorithm that is computationally not intensive and produces uniformly distributed null matrices with fixed row and column totals. Thanks to its efficiency, our method can be applied even to very large matrices (>10 8 cells) using ordinary personal computers. To remain with the baseball analogy, we named this procedure the ‘Curveball algorithm’, as it approaches the issue from an unexpected direction. Intuition Let us imagine that a group of children meets to exchange baseball cards. We assume that all cards have the same value, so that a fair trade is one in which one card is given for one card received, and that no one is interested in holding duplicate cards. This scenario may be represented by a matrix with rows corresponding to children and columns corresponding to cards. Each cell in that matrix will be filled (that is, equal to 1) if the child of the respective row owns the card of the respective column, and empty (that is, equal to 0) if the child does not. Now imagine that two children, after comparing their decks of cards, make a trade according to the above rules, that is, a card is given for one card received, and no trade that leads a child to own more than one card per type is made. Let us assume that some trades are feasible, that is, there are some pairs of children where one of the two owns some cards not owned by the other and vice versa, and let us have a look at the situation after a few of the possible trades have taken place. No card has been created or destroyed during the whole trade process. Because of the fair-trade rule, the number of cards owned by each child has not changed. And because of the one-card-per-type rule, the number of children owning a particular card has also not changed. Thus, if we put back children and cards in rows and column, we will obtain a matrix with a configuration different from the starting one but with the same row and column totals. Description of the algorithm Functioning of the Curveball algorithm is illustrated in Fig. 1 . For the sake of clarity, in the following example, we will refer to a species per site matrix, but the algorithm can be applied to any binary matrix. We call sites A1, A2, … An, and species Sp1, Sp2, … Spn. If the number of species is higher or equal than that of sites, a set of lists of all the species occurring in each site is created ( a ). Then, two lists are extracted at random from this set ( b ). Throughout the text, we will refer to this kind of process using the term ‘pair extraction’. Suppose we have extracted sites A2 and A3. The two lists of species (A2 and A3) are compared to identify the set of species present in A2 but not in A3 (A 2-3 ) and the set of species present in A3 but not in A2 (A 3-2 ) ( c ). In our example, A 2-3 has one element, whereas A 3-2 has two elements. Thus one species of A3 extracted at random from the set A 3-2 is ‘traded’ with the one species of A2 belonging to the set A 2-3 ( d ). In general, for any random pair of lists, a certain number of elements exclusive of a list are traded with an equal number of elements exclusive of the other list. The number of trades for each pair of lists will vary randomly from 0 to n , where n is the size of the smaller of the two sets of exclusive elements. 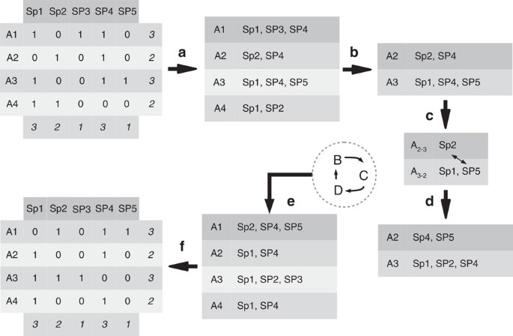Figure 1: Functioning of the Curveball algorithm. Given a species per site binary matrix, a set including the lists of all species (columns) occurring in each site (rows) is created (a). Two lists are extracted at random from this set (b). The two lists are compared to identify the set of species occurring in one list but not in the other and vice versa (A2-3and A3-2) (c). A2-3has one element, whereas A3-2has two elements. Thus one species of A3 extracted at random from the set A3-2is ‘traded’ with the one species of A2 belonging to the set A2-3(d). After the steps (btod) have been reiterated for a certain number of times (e), the randomized set of species per site lists is used to recompile the presence-absence matrix (f). Figure 1: Functioning of the Curveball algorithm. Given a species per site binary matrix, a set including the lists of all species (columns) occurring in each site (rows) is created ( a ). Two lists are extracted at random from this set ( b ). The two lists are compared to identify the set of species occurring in one list but not in the other and vice versa (A 2-3 and A 3-2 ) ( c ). A 2-3 has one element, whereas A 3-2 has two elements. Thus one species of A3 extracted at random from the set A 3-2 is ‘traded’ with the one species of A2 belonging to the set A 2-3 ( d ). After the steps ( b to d ) have been reiterated for a certain number of times ( e ), the randomized set of species per site lists is used to recompile the presence-absence matrix ( f ). Full size image This mechanism makes it possible to randomize the original set of species–site associations without altering the total numbers of species and sites in the newly generated lists. After the steps b to d have been reiterated for a certain number of times ( e ), the randomized set of species lists is used to recompile the presence-absence matrix ( f ). If the number of species is lower than that of the sites, the procedure is the same, with the only difference that pair extractions are performed on a set including the lists of all sites where each species occurs. Two examples of implementation of the algorithm in Python programming language ( www.python.org ) and R ( www.r-project.org ) are available in Supplementary Software 1–5 . Uniform distribution of null matrices Ideally the performance of a randomization algorithm should be measured by assessing how extensively it explores the universe of possible matrix configurations that satisfy the requirement of fixed row and column totals. In other words, the algorithm should not show any preference for particular matrix configurations [13] . We investigated the robustness of the Curveball algorithm towards this issue by using the same theoretical and empirical approaches that have been already used to test swap algorithms [13] , [14] . The five matrices shown in Fig. 2 represent all the possible configurations of a 3 × 3 matrix with row column totals both equal to [1-2-1]. Starting from any of these five matrices, an unbiased algorithm should generate null matrices corresponding to the five different configurations with the same frequency. 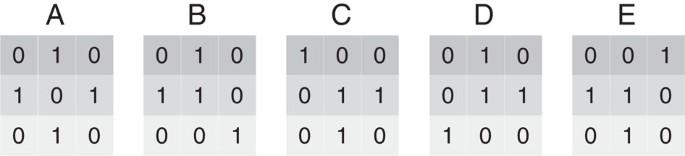Figure 2: The five possible configurations of a presence-absence matrix with both row and column totals equal to [1, 2, 1]. . Figure 2: The five possible configurations of a presence-absence matrix with both row and column totals equal to [1, 2, 1]. . Full size image The transition matrix of the Curveball algorithm for this set of matrices, which expresses the probability that a single pair extraction will lead from a matrix configuration to another, is reported in Table 1 . The eigenvector solution provides the expected frequencies of the different matrices produced by performing several pair extractions ( Table 2 ), and demonstrates that the Curveball algorithm ensures uniformity in the distribution of null matrices A–E. 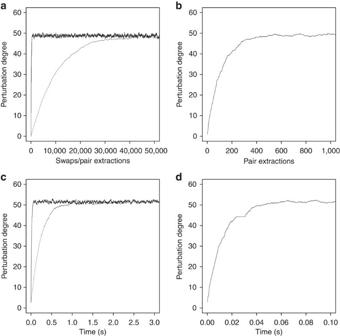Figure 3: Comparisons between computational demand of swaps and pair extractions necessary to perturb a 100 × 100 random matrix. Perturbation is measured as the percentage of cells differing from the corresponding ones of the original matrix. (a) Relationship between number of performed pair extractions (continuous line) and swaps (dotted line), and the corresponding matrix perturbation degree; (b) relationship between number of performed pair extractions and the corresponding matrix perturbation degree; (c) relationships between the computational time (in seconds) of pair extractions (continuous line) and swaps (dotted line), and the corresponding matrix perturbation degree; (d) relationships between the computational time (in seconds) of pair extractions and the corresponding matrix perturbation degree. Of note, as few as five pair extractions are sufficient to reach the uniform distribution (see Table 3 , which reports the 5th power of the transition matrix). Table 1 Transition rate matrix of the five possible configurations shown in Fig. 2 for the Curveball algorithm. Full size table Table 2 The 25th power of the transition rate matrix reported in Table 1 . Full size table Table 3 The 5th power of the transition rate matrix reported in Table 1 . Full size table It should be highlighted that the transition probabilities reported in Table 1 refer to any attempted pair extraction, and not only to those leading to some trade of elements, which is consistent with the formulation of the Curveball algorithm (and with the basic idea behind the trial-swap method [14] ). However, this issue, which is of central importance for swap algorithms [14] , does not affect the Curveball algorithm, as the convergence to the uniform distribution is ensured even in the case when only pair extractions leading to some trade of elements are considered ( Supplementary Tables 1 and 2 ). To provide empirical support to the theoretical expectations, we used the Curveball algorithm to generate a set of 10,000 null matrices for each one of the five configurations of Fig. 1 . Then we tested in each set if the distribution frequency of the five possible configurations was significantly different from 1:1:1:1:1. In all sets we observed a distribution frequency of null matrices statistically not different from the desired uniform distribution (average P -value of χ 2 tests=0.73, standard error=0.08). Additional evidence that the Curveball algorithm samples different null matrices with frequencies not deviating from an unbiased uniform distribution is provided in Supplementary Note 1 . Computational demand of the Curveball algorithm We performed a simple test to compare the difference in terms of computational effort between the Curveball algorithm and the swap methods. For this we compared the number of pair extractions and the number of swap attempts necessary to maximally perturb a matrix, that is, to reach a situation where the percentage of matrix cells in a different position with respect to the starting configuration remains stable when new swap attempts/pair extractions are performed. To this purpose we used a moderately large random matrix of 100 rows × 100 columns that we created by filling cells with 0 and 1 with the same probability. Then we conducted two separate analyses by performing, respectively, one million pair extractions and one million swap attempts on that matrix. In both analyses, we measured at each step the percentage of cells differing from the corresponding ones in the original matrix. After a certain number of pair extractions and swaps, the average percentage of cells with different values from the original configuration became stable (with a value around 50%, Fig. 3a ). To reach this plateau, about 50,000 swap attempts were necessary, which is consistent with the number recommended by recent work [17] , [22] . Crucially, the same value was reached by the Curveball algorithm after less than 200 iterations ( Fig. 3b ). Figure 3: Comparisons between computational demand of swaps and pair extractions necessary to perturb a 100 × 100 random matrix. Perturbation is measured as the percentage of cells differing from the corresponding ones of the original matrix. ( a ) Relationship between number of performed pair extractions (continuous line) and swaps (dotted line), and the corresponding matrix perturbation degree; ( b ) relationship between number of performed pair extractions and the corresponding matrix perturbation degree; ( c ) relationships between the computational time (in seconds) of pair extractions (continuous line) and swaps (dotted line), and the corresponding matrix perturbation degree; ( d ) relationships between the computational time (in seconds) of pair extractions and the corresponding matrix perturbation degree. Full size image This does not necessary imply that the difference between the two algorithms, in terms of computational effort, scales accordingly, as comparing and recombining the species composition of two areas is more complex than evaluating and swapping a 2 × 2 matrix. Moreover, the amount of data processed by a swap attempt is constant, whereas that processed by a pair extraction is not. To investigate this aspect, we replicated the above test by recording the time necessary to reach the maximum matrix perturbation using, alternatively, swaps and pair extractions. We recorded only the time necessary to attempt single swaps (that is, the random selection and, if possible, the swap of a 2 × 2 submatrix), and single pair extractions (that is, the random extraction of two species-area lists, the comparison of the two lists and, if possible, the random exchange of some not-shared elements). We performed this test on a quad-core (Intel Xeon E5-2630 @ 2.30 GHz) workstation hosting a 64-bit Linux OS. Using swap attempts, the time required to reach the maximum perturbation was around 1 s ( Fig. 3c ). Using pair extractions, the maximum perturbation was reached about twenty times faster (~0.05 s, see Fig. 3d ). Another important aspect to be considered is that matrix fill affects significantly swap algorithms, as the more it deviates from 0.5, the lower is the probability that a swap attempt will be successful. Conversely, the Curveball algorithm should be much less affected, due to the fact that it focuses only on matrix presences. However, we investigated this issue empirically, by replicating the above experiment on six different random matrices of 100 rows × 100 columns with different fill values (respectively, 10%, 30%, 50%, 70%, 90%). As expected, matrix fill significantly affected the number of swap attempts necessary to maximally perturb the matrix. In particular, a large number of swap attempts (~100,000) was necessary for the least- and the most-filled matrices ( Fig. 4a ). By contrast, the differences in matrix fill did not affect the performance of the Curveball algorithm ( Fig. 4b ). Analogous patterns were observable when computational time (measured as described above) was compared with matrix perturbation ( Fig. 4c,d ). Thus, pair extractions made it possible to reach the maximum perturbation degree of both the most (90%) and the least (10%) filled matrix about 70 times faster than swap attempts did. Noteworthy, in all cases, the maximum percentage of matrix perturbation reached using pair extractions was always higher than that reached using swaps. 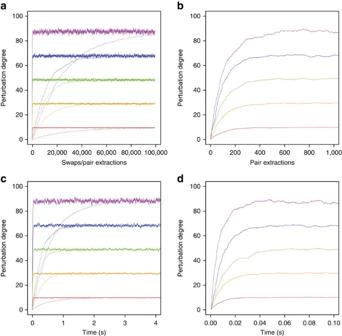Figure 4: Comparisons between computational demand of pair extractions and swaps necessary to perturb five 100 × 100 random matrices with different fill values. Perturbation is measured as the percentage of cells differing from the corresponding ones of the original matrix. (a) Relationship between number of performed pair extractions (continuous lines) and swaps (dotted lines), and the corresponding matrix perturbation degree; (b) relationship between number of performed pair extractions and the corresponding matrix perturbation degree; (c) relationships between the computational time (in seconds) of pair extractions (continuous lines) and swaps (dotted lines), and the corresponding matrix perturbation degree; (d) relationships between the computational time (in seconds) of pair extractions and the corresponding matrix perturbation degree. Colours indicate different fill values (magenta=10%; blue=30%; green=50%; orange=70%; red=90%). Figure 4: Comparisons between computational demand of pair extractions and swaps necessary to perturb five 100 × 100 random matrices with different fill values. Perturbation is measured as the percentage of cells differing from the corresponding ones of the original matrix. ( a ) Relationship between number of performed pair extractions (continuous lines) and swaps (dotted lines), and the corresponding matrix perturbation degree; ( b ) relationship between number of performed pair extractions and the corresponding matrix perturbation degree; ( c ) relationships between the computational time (in seconds) of pair extractions (continuous lines) and swaps (dotted lines), and the corresponding matrix perturbation degree; ( d ) relationships between the computational time (in seconds) of pair extractions and the corresponding matrix perturbation degree. Colours indicate different fill values (magenta=10%; blue=30%; green=50%; orange=70%; red=90%). Full size image However, the difference in performance between the Curveball algorithm and swap methods is not surprising. Let us imagine a matrix of R rows and C columns having only one checkerboard. A matrix of this kind admits only one alternative configuration. The probability to find this sole configuration by extracting 2 × 2 submatrices is equal to 1/( R 2 × C 2 ). Conversely, the probability to find it by using pair extractions is 1/ R 2 (if R < C ) or 1/ C 2 (if R > C ). In general the Curveball algorithm perturbs the matrix in most of the pair extractions, whereas the swap methods have to check several submatrices to obtain the same effect. 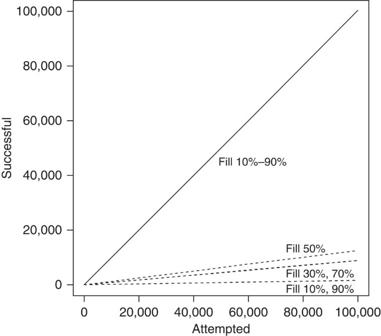Figure 5: Relationship between the number of attempted pair extractions and swaps and the corresponding number of successful ones for five 100 × 100 random matrices with different fill values. Continuous lines correspond to pair extractions, whereas dotted lines correspond to swaps. All the five lines reporting the relationships for pair extractions are almost perfectly overlapping. A nearly perfect overlap is also observed in the lines reporting the relationships for swaps for the two pairs of matrices with respective fill equal to 10 and 90%, and 30 and 70%. Figure 5 shows the relationship between the number of attempted swaps/pair extractions and the corresponding number of successful ones (that is those producing some change on the matrix) for matrices of various fill. Independent of matrix fill, almost each pair extraction produces some modification to the matrix. By contrast, for a 50% filled matrix, approximately eight random attempts are necessary to successfully perform a swap. This number increases symmetrically for less- and more-filled matrices (~10 for a 30% and a 70% filled matrix, and ~60 for a 10% and a 90% filled matrix). Figure 5: Relationship between the number of attempted pair extractions and swaps and the corresponding number of successful ones for five 100 × 100 random matrices with different fill values. Continuous lines correspond to pair extractions, whereas dotted lines correspond to swaps. All the five lines reporting the relationships for pair extractions are almost perfectly overlapping. A nearly perfect overlap is also observed in the lines reporting the relationships for swaps for the two pairs of matrices with respective fill equal to 10 and 90%, and 30 and 70%. Full size image The statistical challenge that originated this study has interested ecologists for more than 30 years [4] . Exploring the universe of different configurations of matrices with fixed row and column sums has also several applications in other scientific fields, including neurophysiology (in the study of multivariate binary time series), sociology (in the analysis of affiliation matrices) and psychometrics (in item response theory) [21] . Yet, most of the solutions that have been proposed so far present major drawbacks. Unbiased algorithms are computationally very intensive and therefore slow, whereas faster algorithms do not ensure that different null matrices are generated with equal frequencies, which may affect result robustness [14] . Another limitation is that most of the available methods cannot be easily used for very large matrices. What makes these algorithms slow is that they require a very large number of iterations to properly randomize the original matrix. A recent study demonstrated that more than 50,000 swaps are necessary to prevent the occurrence of type I errors in a matrix of average size, and that, for large matrices, many more swaps are needed [17] . The same authors also suggest that, if the data set under examination is particularly large, the analysis should be repeated by progressively increasing the number of swaps until the P -value stabilizes. In common ecological analyses, a standard number of null matrices to assess the significance of a given pattern is 1,000, and in macroecological studies, it is quite common to investigate patterns in tens (sometimes hundreds) of large matrices [23] . Thus, to evaluate the significance of ecological patterns in a set of 100 matrices, a total of 5 × 10 9 swaps is needed. This is quite a large number, even for modern calculators, so that the task would inevitably be time consuming. By contrast, the number of pair extractions the Curveball algorithm requires to obtain an unbiased sample of null matrices is moderately small even for large matrices ( Supplementary Fig. 1 and Supplementary Note 2 ). However, the main issue connected to swap algorithms is that they do not ensure robust results for large matrices unless the number of swaps is raised to a number that makes computation itself rather impractical. To provide support to their observations, Fayle and Manica [17] performed some tests on artificial matrices of 900 rows × 400 columns to simulate the maximum size of matrices ever used in a null model analysis. A matrix of this size is arguably large from an ecological perspective. However, the increasing data availability for both geographical distribution and ecological networks offers new possibilities to investigate ecological patterns at a very large scale and/or at a very high resolution [24] . This makes it likely that the use of matrices even larger than the above-mentioned ones will become quite common in the next few years. For this, better performing algorithms are needed. In this paper we propose a solution to a long-debated methodological puzzle. All the tests we performed suggest that the Curveball algorithm is more efficient than most available tools. Using a simple R function (which is provided in Supplementary Software 5 ), the Curveball algorithm was able to randomize a 10 4 × 10 4 matrix in less than 10 seconds on a budget notebook equipped with a dual core processor (Intel Core i3-370M @ 2.40 GHz) running a 64-bit Linux OS. The same task required almost 30 min when using the independent swap method (with the function randomizeMatrix of the package ‘picante’ [25] ) and setting the number of swaps to the recommended value of twice the number of presences in the matrix multiplied by the number of attempts necessary to successfully perform a swap [14] (as the matrix was approximately 50% filled, we used our estimate of eight attempts per successful swap). Despite the fact that the logic behind the Curveball algorithm and its implementation are quite far from swap methods, the two approaches are in a certain way closely related. In practice, what the Curveball algorithm does is (1) to identify in a single step all the possible swaps between a pair of matrix rows (or columns) and (2) to perform any of them with a random probability. The first aspect makes the algorithm efficient, whereas the second makes it robust towards unequal sampling of random matrices. Although we are convinced ours will not be the last word on the subject, we hope that the principles of our approach will be useful for future research, orienting ecologists’ efforts more on the information the data convey, rather than on the way they are distributed in a matrix. How to cite this article: Strona, G. et al. A fast and unbiased procedure to randomize ecological binary matrices with fixed row and column totals. Nat. Commun. 5:4114 doi: 10.1038/ncomms5114 (2014).